Ice as a protocellular medium for RNA replication A crucial transition in the origin of life was the emergence of an informational polymer capable of self-replication and its compartmentalization within protocellular structures. We show that the physicochemical properties of ice, a simple medium widespread on a temperate early Earth, could have mediated this transition prior to the advent of membraneous protocells. Ice not only promotes the activity of an RNA polymerase ribozyme but also protects it from hydrolytic degradation, enabling the synthesis of exceptionally long replication products. Ice furthermore relieves the dependence of RNA replication on prebiotically implausible substrate concentrations, while providing quasicellular compartmentalization within the intricate microstructure of the eutectic phase. Eutectic ice phases had previously been shown to promote the de novo synthesis of nucleotide precursors, as well as the condensation of activated nucleotides into random RNA oligomers. Our results support a wider role for ice as a predisposed environment, promoting all the steps from prebiotic synthesis to the emergence of RNA self-replication and precellular Darwinian evolution. A critical event in the origin of life is thought to have been the emergence of a polymer capable of self-replication, mutation and hence evolution towards more efficient self-replication. A substantial body of evidence, as formulated in the 'RNA world' hypothesis, supports a central role for RNA in this process [1] . Supporting evidence includes key aspects of modern metabolism (such as nucleotide cofactors), gene expression (splicing, riboswitches) and translation, which involve RNA in both informational and catalytic roles and may thus represent relics from an 'RNA world' [1] , [2] . The adaptability of RNA is further revealed by the evolution of novel receptors (aptamers) and enzymes (ribozymes) by in vitro selection from pools of random RNA oligomers [3] . The recent discovery of an efficient prebiotic synthetic route to the pyrimidine ribonucleotides further strengthens the case for RNA's central role in abiogenesis [4] . However, despite its astonishing catalytic and structural versatility, RNA would seem to be a questionable choice as a primordial genetic material, as its vicinal 2′-OH renders it susceptible to degradation by nucleophilic cleavage of the 3′-phosphodiester bond [5] . Because of this inherent fragility under any but the most benign geochemical settings, a self-replicating RNA could only have emerged in a particular environment that enhanced RNA stability while allowing RNA replication. Such an environment ideally would also have provided some form of molecular confinement or colocalization of the replicase and its 'offspring'. This diffusion limitation is a prerequisite for Darwinian evolution [6] , because it averts dissipation of the replicase genotype by fruitless replication of unrelated (and most likely inactive) RNA sequences, and curbs the rise of fast-replicating RNA parasites [7] . Although a range of structured environments, including micelles, membraneous vesicles, porous rocks or even aerosol droplets [8] , [9] , [10] , [11] , [12] , have been proposed as protocellular media capable of providing compartmentalization, their ability to support RNA replication and protect RNA from degradation is unclear. In this study, we show that ice, a simple medium likely to have been widespread on the early Earth, can provide a propitious environment for RNA self-replication and evolution. Examining the in-ice activity of the Round-18 (R18) RNA polymerase ribozyme [13] —the best available 'Doppelganger' [14] of a primordial replicase—as a model system, we find that ice not only supports high-fidelity RNA replication but also greatly stabilizes the RNA polymerase ribozyme, enabling extended RNA replication. Furthermore, we find that ice relieves the dependence of ribozyme activity on prebiotically implausible solute and substrate concentrations, and enables RNA replication from solute concentrations found in present day freshwater sources. Finally, we show that in ices formed from such dilute starting mixtures, the topological structure of the eutectic phase undergoes dramatic changes, which slow down ribozyme diffusion by more than three orders of magnitude, providing de facto compartmentalization of RNA replication. Ice supports enzymatic RNA replication by a ribozyme When an aqueous solution of ions or other solutes is cooled to below its freezing point, a biphasic system is formed, whereby solutes are excluded from the growing ice crystals and are concentrated in an interstitial liquid brine, the eutectic phase. Ice crystal growth causes the progressive dehydration and concentration of solutes [15] , accelerating many chemical reactions, notably the formation of RNA oligomers by non-enzymatic polymerization of activated nucleotides [16] , [17] , [18] , [19] . Thus, ice has the potential to provide, in situ , starting materials for prebiotic RNA evolution. This prompted us to investigate the potential of ice to promote the next stage of RNA-based evolution: the emergence of RNA self-replication. The R18 RNA polymerase ribozyme [13] construct ( Fig. 1a ) studied herein, although presumably more complex than the earliest replicators (which might have been simpler ribozyme polymerases or ligases [20] ), was the only ribozyme with substantial RNA polymerase activity, and thus represented the best available model system for studying RNA-catalysed RNA replication. 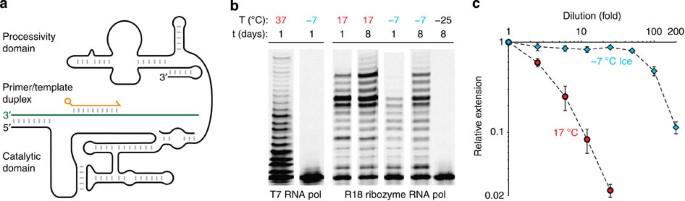Figure 1: RNA polymerase activity at ambient temperature and in ice. (a) Schematic of the polymerase ribozyme. The catalytic and processivity domains of the ribozyme (black) are depicted surrounding the primer-template duplex. The 5′ terminus of this ribozyme variant is designed to hybridize on the RNA template (green) upstream of the primer (orange) (Supplementary Fig. S1). (b) Fluorescent primer extension reactions using a proteinaceous polymerase (T7 RNA polymerase) and the ribozyme RNA polymerase at ambient temperatures (red) and in ice (blue), resolved by denaturing gel electrophoresis. (c) Average primer extension in diluted reactions after 7 days at 17 °C (red circles) or in ice at −7 °C (blue diamonds) relative to undiluted reactions at these temperatures (means ± s.e.m.,n=3). Figure 1: RNA polymerase activity at ambient temperature and in ice. ( a ) Schematic of the polymerase ribozyme. The catalytic and processivity domains of the ribozyme (black) are depicted surrounding the primer-template duplex. The 5′ terminus of this ribozyme variant is designed to hybridize on the RNA template (green) upstream of the primer (orange) ( Supplementary Fig. S1 ). ( b ) Fluorescent primer extension reactions using a proteinaceous polymerase (T7 RNA polymerase) and the ribozyme RNA polymerase at ambient temperatures (red) and in ice (blue), resolved by denaturing gel electrophoresis. ( c ) Average primer extension in diluted reactions after 7 days at 17 °C (red circles) or in ice at −7 °C (blue diamonds) relative to undiluted reactions at these temperatures (means ± s.e.m., n =3). Full size image However, ice did not seem to be an auspicious medium for RNA replication. Low temperatures can negatively affect macromolecular catalysis in multiple ways, which impinge upon both chemistry and catalyst – for example, by stabilizing alternative secondary structures [21] , by cold denaturation [22] , and by affecting molecular motions and conformational transitions essential for catalysis and template translocation by polymerases [23] . Indeed, although a simple ligase ribozyme has been reported to retain some activity when frozen [24] , freezing completely abolished the activity of the T7 RNA polymerase ( Fig. 1b ). However, we found that the R18 RNA polymerase ribozyme [13] ( Fig. 1a , Supplementary Fig. S1 ) not only retained its RNA polymerase activity in ice ( Fig. 1b ) but was, in fact, more active in ice than in super cooled solutions of the same temperature (−7 °C) ( Supplementary Fig. S2 ). Further cooling (to −25 °C) of the frozen reaction mixture towards the eutectic point abolished activity, indicating that a liquid brine phase is required for polymerase activity. Ribozyme polymerase activity in ice, although slower, persisted for much longer. Although reactions at ambient temperatures yielded only modest additional extension after 2 days, replication activity in ice continued for days and weeks, allowing it to 'catch-up', that is, synthesize equally long extension products after incubation for 8 days. Thus, although proteinaceous RNA polymerases are inactivated by freezing, ribozyme-catalysed RNA replication can proceed within the eutectic phase of ice, and with unexpectedly high efficiency. Freezing enables RNA replication from highly dilute solutions Freezing the reactions made ribozyme polymerase activity remarkably robust to depletion of crucial solutes. High concentrations of ribonucleotide triphosphates and magnesium salts (MgCl 2 ) are both essential for ribozyme activity [13] ; reducing them by dilution resulted in a sharp decrease in ribozyme activity in solution (both at ambient temperature (17 °C) or in a super cooled solution (−7 °C)) ( Supplementary Fig. S2 ). In contrast, RNA polymerase ribozyme activity in ice remained unchanged, even after dilution of reactions by 50-fold, and persisted after dilutions of up to 200-fold ( Fig. 1c ). Owing to the equilibrium between the ice phase and the eutectic phase, ice crystal growth only ceases when a certain solute concentration has been reached in the eutectic phase [15] . Thus, more dilute starting conditions do not lead to a more dilute eutectic phase but rather reduce its volume until the same equilibrium concentration is reached. From dilute starting reactions, we estimate the concentration enhancement to be >200-fold ( Supplementary Note ), enabling near optimal RNA replication activity from micromolar nucleotide concentrations and from magnesium ion (Mg 2+ ) concentrations typically found in present day freshwater sources. Ion identity affects in-ice RNA replicase activity Positive counterions such as magnesium (Mg 2+ ) are critical cofactors of ribozyme structure and activity. Indeed, the cationic requirements of the class I RNA ligase ribozyme (the catalytic core of the RNA polymerase ribozyme [25] ) have been investigated in detail and its activity has been found to be strictly dependent on Mg 2+ , with all other cations (including Mn 2+ ) strongly inhibitory [26] . However, in contrast to the well-studied functional roles of positive counterions such as Mg 2+ , the influence of negative counterions was not considered previously. We therefore replaced the main negative counterion chloride (Cl − ) with a range of alternative counterions (SO 4 2− , CH 3 COO − , Br − , NO 3 − ), while maintaining equimolar levels of Mg 2+ , and studied their effect on ribozyme polymerase activity both in ice and at ambient temperature. The identity of the negative counterion exerted limited influence on ribozyme activity at 17 °C, but affected ribozyme polymerase activity noticeably in ice ( Fig. 2a ). Although some counterions were inhibitory, replacement of Cl − with sulphate (SO 4 2− ) substantially enhanced in-ice polymerase ribozyme activity, despite inhibiting it in solution. Intriguingly, ranking of counterion effects in ice (but not at ambient temperature or in supercooled solutions) followed the Hofmeister series [27] . The more chaotropic anions such as nitrate and bromide reduced in-ice extension, whereas sulphate (SO 4 2− ), a kosmotropic anion, substantially enhanced in-ice polymerase ribozyme activity. 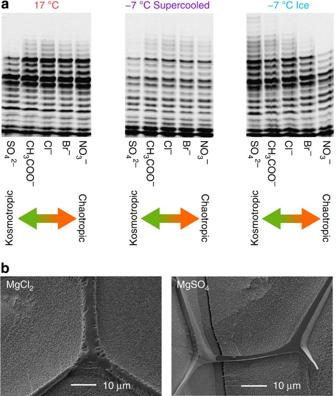Figure 2: Solute influence on ribozyme activity and ice structure. (a) Primer extension in reactions (8 days, 4 mM of each ribonucleotide triphosphate) in which the Cl−counterion of magnesium was replaced with a range of other counterions, displayed in the order of position in the Hofmeister series. (b) The eutectic phase in ice formed at −7 °C from undiluted extension reactions with MgCl2or MgSO4, imaged by freeze-fracture SEM. The raised veins of the eutectic phase are on average visibly narrower in ice formed with equimolar amounts of MgSO4. Figure 2: Solute influence on ribozyme activity and ice structure. ( a ) Primer extension in reactions (8 days, 4 mM of each ribonucleotide triphosphate) in which the Cl − counterion of magnesium was replaced with a range of other counterions, displayed in the order of position in the Hofmeister series. ( b ) The eutectic phase in ice formed at −7 °C from undiluted extension reactions with MgCl 2 or MgSO 4 , imaged by freeze-fracture SEM. The raised veins of the eutectic phase are on average visibly narrower in ice formed with equimolar amounts of MgSO 4 . Full size image Hofmeister effects on macromolecular function are well known and ubiquitous [28] . However, the restriction of the effects to in-ice polymerase activity argues against temperature-dependent interactions of the negative counterion with the ribozyme or its hydration shell; rather, it suggests indirect effects on water structure [29] and ice crystal growth. Indeed, the eutectic point of MgSO 4 is −4 °C [30] , nearly 30 °C higher than that of MgCl 2 (−33 °C). Although attenuated by the presence of other solutes in the reaction, the higher eutectic point and consequently much weaker depression of the freezing temperature by equimolar amounts of MgSO 4 , compared with MgCl 2 , would result in more extensive freezing, affecting the eutectic phase microstructure. Scanning electron microscopy (SEM) imaging of freeze-fractured eutectic ice phases ( Fig. 2b ) indeed suggests a decreased eutectic phase volume in MgSO 4 ices, and consequently a presumably increased concentration effect upon eutectic phase formation. Ice stabilizes the ribozyme and prolongs its activity Having established that ice was able to support ribozyme-catalysed RNA replication, we sought to investigate whether it might also increase RNA stability because of the reduced temperature and water activity in the eutectic phase. The dependence of the RNA polymerase ribozyme on high Mg 2+ concentrations for optimal activity accelerates the hydrolysis of its RNA backbone [31] , limiting its half-life to <52 h at 17 °C. However, at −7 °C in ice, its half-life was increased to >16 days ( Fig. 3 ). We asked whether this increase in stability would translate into prolonged activity and longer extension products. We found that, whereas ribozyme activity at ambient temperatures ceased after a few days (extending a primer by up to 16 nucleotides), ribozyme polymerase activity in ice continued for weeks, yielding extension products 23 nucleotides long after 25 days. Replacing the Cl − counterion with SO 4 2− allowed RNA replication products up to 32 nucleotides long to be generated in ice ( Fig. 4a ). 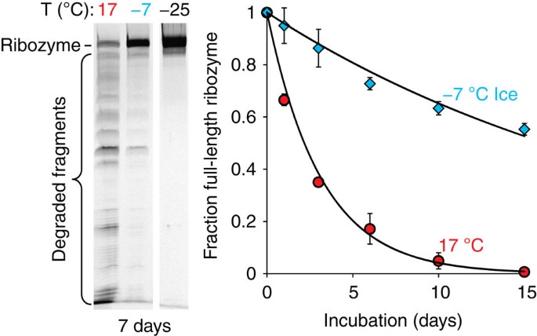Figure 3: Enhanced in-ice ribozyme stability. Degradation of 5′-fluorescein-labelled RNA polymerase ribozyme in extension buffer (200 mM Mg2+) for 7 days (left panel) and as a function of time (right panel) at 17 °C (red circles) or in ice at −7 °C (blue diamonds) (means ± s.d.,n=3). Exponential decay functions were fit to the data, suggesting decay constants of 0.319 (17 °C;R2=0.9945) and 0.043 (−7 °C;R2=0.973) per day. Figure 3: Enhanced in-ice ribozyme stability. Degradation of 5′-fluorescein-labelled RNA polymerase ribozyme in extension buffer (200 mM Mg 2+ ) for 7 days (left panel) and as a function of time (right panel) at 17 °C (red circles) or in ice at −7 °C (blue diamonds) (means ± s.d., n =3). Exponential decay functions were fit to the data, suggesting decay constants of 0.319 (17 °C; R 2 =0.9945) and 0.043 (−7 °C; R 2 =0.973) per day. 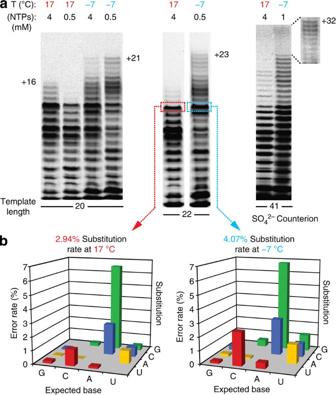Figure 4: In-ice RNA replication and fidelity. (a) Enhanced RNA primer extension in ice. Shown are fluorescent primer extension reactions after 25 days of incubation, resolved by denaturing gel electrophoresis. Extension in ice reaches 23 nucleotides (in standard MgCl2extension buffer) or 32 nucleotides on a longer template in MgSO4extension buffer (right panel, with inset showing high-sensitivity scan of indicated area) using reduced ribonucleotide triphosphate concentrations (NTPs) (Supplementary Note). (b) High-throughput sequencing of 12 nucleotide extension products reveals comparable replication fidelities and error spectra in solution and in ice. Full size image Figure 4: In-ice RNA replication and fidelity. ( a ) Enhanced RNA primer extension in ice. Shown are fluorescent primer extension reactions after 25 days of incubation, resolved by denaturing gel electrophoresis. Extension in ice reaches 23 nucleotides (in standard MgCl 2 extension buffer) or 32 nucleotides on a longer template in MgSO 4 extension buffer (right panel, with inset showing high-sensitivity scan of indicated area) using reduced ribonucleotide triphosphate concentrations (NTPs) ( Supplementary Note ). ( b ) High-throughput sequencing of 12 nucleotide extension products reveals comparable replication fidelities and error spectra in solution and in ice. Full size image Replication proceeds with high fidelity in ice Replication must proceed with a certain degree of accuracy to avoid an 'error catastrophe' and irreversible corruption of the encoded genetic information [32] . Temperature influences the strength of molecular interactions and is known to affect the substrate discrimination and fidelity of proteinaceous polymerases [33] . Indeed, the recognition specificity of the hairpin ribozyme was found to be greatly reduced at subzero temperatures [24] . We therefore wondered whether the enhanced RNA replication in ice had been achieved at the expense of replication fidelity. We determined ribozyme error rates by high-throughput sequencing of >3,000 extension products from ambient temperature (17 °C) and in-ice (−7 °C) reactions. These provided values for RNA polymerase ribozyme misincorporation fidelity at ambient temperatures (97.1%) in excellent agreement with previous estimates (96.7% (ref. 13 )) and yielded a very similar value for ribozyme fidelity in ice (95.9%) ( Fig. 4b ). Furthermore, detailed inspection of the error spectrum and sequence dependency revealed closely matching mutation signatures and hotspots at both temperatures ( Supplementary Fig. S3 ), with the only notable difference being an elevated rate of deletion mutations in ice (2.4%) compared with ambient temperatures (0.8%). These findings confirm that replication fidelity is maintained when the RNA polymerase ribozyme operates at subzero temperatures. Thus, eutectic ice phases are able to support and enhance RNA replication without compromising replication fidelity. Ice compartmentalizes ribozyme catalysis Compartmentalization and colocalization of a replicase and its offspring is a prerequisite for Darwinian evolution [6] . Thus, RNA replication in a medium does not per se imply a capacity of that medium to support RNA evolution. Elegant in silico experiments [7] have previously shown that diffusion limitation can provide functional colocalization and compartmentalization and support replicase evolution by ensuring kin selection through reciprocal altruism. Diffusion restriction links phenotype and genotype and allows evolution, while simultaneously limiting the spread of parasitic RNAs. Ice is highly structured at the microscale, with the eutectic phase forming a complicated network of brine-filled spaces and channels interspersed between the ice crystals. We questioned whether such lattice structures could be shaped to effectively restrict ribozyme diffusion and afford a form of quasicellular compartmentalization. We sought to detect this beneficial trait using a sensitive assay for ribozyme diffusion through the ice. To this end, we randomly dispersed beads decorated with RNA primer-template duplexes within an ice column of defined volume as a 'scoring grid' ( Fig. 5a , Supplementary Fig. S4 ) and analysed diffusion of active RNA polymerase ribozyme molecules through the ice column by counting ribozyme bead encounters using fluorescence-activated cell sorting. Not unexpectedly, our results show a dramatic restriction of ribozyme diffusion through ice, with ribozyme requiring over a week to reach 70% of the beads ( Supplementary Fig. S4 ). Furthermore, we found that ribozyme diffusion was decreased further in ice formed from more dilute starting mixtures ( Fig. 5b,c ), dropping sharply as a function of higher dilutions. 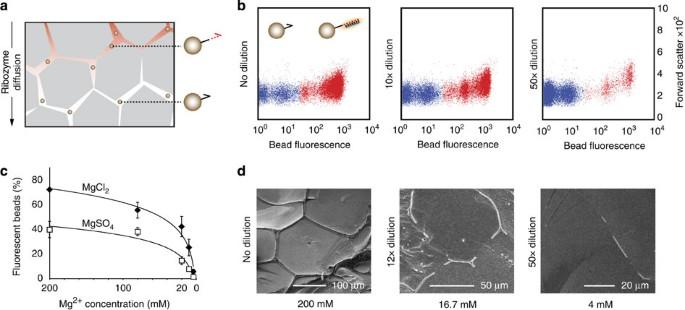Figure 5: Diffusion limitation by ice microstructure. (a) Principle of the in-ice diffusion assay. Ice microstructure limits the exposure of primer-coated 1 μm-diameter beads to diffusing ribozyme; hence, only a subset of the beads experience primer extension (red). (b) Fluorescence-activated cell sorting profiles of beads from different MgCl2ices (after 8 days diffusion). Beads with many extended primers (red) gain fluorescence during processing. (c) The extent of ribozyme diffusion after 8 days (as measured by the percentage of fluorescent beads) through ices with different solute levels and magnesium counterions (filled diamonds, MgCl2; open squares, MgSO4; means ± s.e.m.;n=3). (d) The structure of the eutectic phase in diluted MgCl2reactions, imaged by freeze-fracture SEM. The lighter, raised web of channels represents the eutectic phase. Figure 5: Diffusion limitation by ice microstructure. ( a ) Principle of the in-ice diffusion assay. Ice microstructure limits the exposure of primer-coated 1 μm-diameter beads to diffusing ribozyme; hence, only a subset of the beads experience primer extension (red). ( b ) Fluorescence-activated cell sorting profiles of beads from different MgCl 2 ices (after 8 days diffusion). Beads with many extended primers (red) gain fluorescence during processing. ( c ) The extent of ribozyme diffusion after 8 days (as measured by the percentage of fluorescent beads) through ices with different solute levels and magnesium counterions (filled diamonds, MgCl 2 ; open squares, MgSO 4 ; means ± s.e.m. ; n =3). ( d ) The structure of the eutectic phase in diluted MgCl 2 reactions, imaged by freeze-fracture SEM. The lighter, raised web of channels represents the eutectic phase. Full size image Solute identity affects ice structure and ribozyme activity SEM imaging of freeze-fractured eutectic ice phases revealed a possible physical basis for this effect, as we observed striking changes in eutectic phase volume and topological structure on the progressive reduction of the starting solute concentration ( Fig. 5d ). As adjacent ice crystals fuse, the connectivity of the brine channel network is reduced, yielding a sparse, thin and increasingly fragmented network of brine veins. Ices in which the main negative counterion chloride (Cl − ) is replaced by sulphate (SO 4 2− ) display an even narrower brine vein structure ( Fig. 2b ); this more constricted ice microstructure may account for the enhanced RNA replicase activity ( Fig. 2a ) and the further reduced ribozyme diffusion observed in sulphate ices ( Fig. 5c ). Thus, solute identity and concentration can determine ice microstructure and alter ribozyme replication activity and diffusivity. For ices formed from the most dilute starting mixtures (>50× dilution, [Mg 2+ ]<4 mM), ribozyme diffusivity was over three orders of magnitude lower than in the solution phase ( Fig. 6a , Supplementary Fig. S5 ). 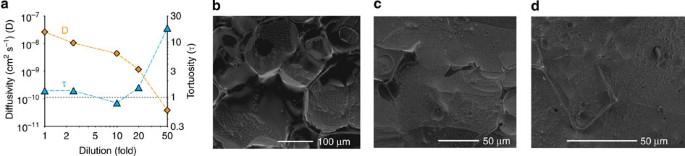Figure 6: Topological transitions in the ice microstructure. (a) The calculated in-ice diffusivity (D, orange diamonds) of ribozyme and the corresponding tortuosity (τ, blue triangles) of the eutectic phase in MgCl2ices (Supplementary Fig. S5). (b–d) Ices formed from undiluted (b), 12-fold diluted (c) and 50-fold diluted (d) extension reactions were flash-frozen in liquid N2to preserve the eutectic phase structure and freeze-fractured, as inFigures 2band5d; however, the samples then underwent prolonged sublimation before gold deposition and SEM imaging. This preferential sublimation of the ice crystals exposes the three-dimensional ultrastructure of the eutectic phase, revealing the prominent sheets of a contiguous eutectic phase in the undiluted reaction (b). Dilution leads to a decrease in the volume of the eutectic phase, manifested by fusion of adjacent ice crystals and shrinking of contiguous sheets of eutectic phase to a network of tubular channels along the vertices of crystals (c), and eventually to sparsely distributed clusters of filamentous tubes (d). Figure 6: Topological transitions in the ice microstructure. ( a ) The calculated in-ice diffusivity (D, orange diamonds) of ribozyme and the corresponding tortuosity ( τ , blue triangles) of the eutectic phase in MgCl 2 ices ( Supplementary Fig. S5 ). ( b – d ) Ices formed from undiluted ( b ), 12-fold diluted ( c ) and 50-fold diluted ( d ) extension reactions were flash-frozen in liquid N 2 to preserve the eutectic phase structure and freeze-fractured, as in Figures 2b and 5d ; however, the samples then underwent prolonged sublimation before gold deposition and SEM imaging. This preferential sublimation of the ice crystals exposes the three-dimensional ultrastructure of the eutectic phase, revealing the prominent sheets of a contiguous eutectic phase in the undiluted reaction ( b ). Dilution leads to a decrease in the volume of the eutectic phase, manifested by fusion of adjacent ice crystals and shrinking of contiguous sheets of eutectic phase to a network of tubular channels along the vertices of crystals ( c ), and eventually to sparsely distributed clusters of filamentous tubes ( d ). Full size image Using the R18 RNA polymerase ribozyme as the best available modern day analogue of a primordial replicase, we have shown that ice has the capacity not only to support but to significantly enhance ribozyme-catalysed RNA replication through substrate and solute concentration and attenuation of replicase degradation. Furthermore, it enables RNA evolution through quasicellular compartmentalization within the eutectic phase. Although the microstructure of the eutectic phase in itself impedes diffusive and convective transport of macromolecules (compared with the solution phase), we observed a striking further drop in diffusivity in ice phases formed from more dilute starting mixtures ( Fig. 6a ). Although at present we cannot rule out surface effects, these drastic reductions in ribozyme diffusivity may be fully rationalized by the decreasing volume and increasing fragmentation of the eutectic phase, as observed by SEM imaging ( Fig. 5d ). The sharp increase in relative path length for ribozyme diffusion (as described by the dimensionless tortuosity ( τ ) parameter ( Fig. 6a )) in the most dilute ices is symptomatic of a breakdown of the connectivity of the brine channel network as a function of starting solute concentration. SEM imaging of partially sublimated ices further illustrates the three-dimensional structure of the eutectic phase and its fragmentation in ices formed from more dilute solutions ( Fig. 6b–d ). To better understand the nature of this topological transition, which was noted previously as a sharp reduction in ice electrical conductivity [34] , we performed in silico simulations of a simple grid-lattice model of in-ice diffusion ( Supplementary Methods ). We sought to model the effects of eutectic phase fragmentation by simulating particle diffusion as random walks through an idealized two-dimensional ice crystal lattice ( Fig. 7a ) while progressively adding blocks to the lattice channels. As fragmentation of the channel network increases, diffusion through the lattice begins to drop sharply ( Fig. 7b ), as seen in ices formed from higher solute dilutions. This transition occurs when the number of blocks and ice crystals approaches parity and correlates with the emergence of compartmentalized grid sectors ( Fig. 7c ). 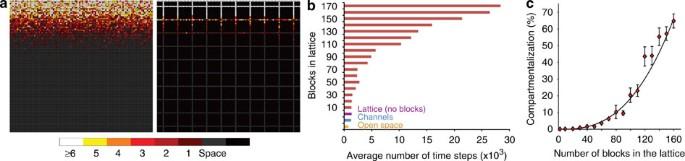Figure 7:In silicomodelling of diffusion through the eutectic phase. (a) Stochastic modelling of ribozyme diffusion in solution (left panel) and in an idealized eutectic lattice (right panel) showing intermediate stages of the diffusion process from ribozymes uniformly distributed at one edge of the experimental space. (b) The average time required for diffusion of 1% of ribozyme particles through the experimental space for an open space ((a), left panel), 1D channels between the edges, and the lattice ((a), right panel) with increasing numbers of blocks (n=50; 30,000 time steps were set as the upper limit per simulation). Introduction of blocks initially has little effect on diffusion, as multiple paths are available through a highly connected system. As the number of blocks rises, connectivity drops, and there is a steep increase not only in the average number of iterations required for 1% of the particles to diffuse through the system but also in the number that cannot cross the experimental space. (c) The percentage of randomly placed static 'beads' inaccessible to diffusing ribozyme—a measure of system compartmentalization—rises steeply as a function of lattice blocks (means ± s.e.m.,n=20). Figure 7: In silico modelling of diffusion through the eutectic phase. ( a ) Stochastic modelling of ribozyme diffusion in solution (left panel) and in an idealized eutectic lattice (right panel) showing intermediate stages of the diffusion process from ribozymes uniformly distributed at one edge of the experimental space. ( b ) The average time required for diffusion of 1% of ribozyme particles through the experimental space for an open space (( a ), left panel), 1D channels between the edges, and the lattice (( a ), right panel) with increasing numbers of blocks ( n =50; 30,000 time steps were set as the upper limit per simulation). Introduction of blocks initially has little effect on diffusion, as multiple paths are available through a highly connected system. As the number of blocks rises, connectivity drops, and there is a steep increase not only in the average number of iterations required for 1% of the particles to diffuse through the system but also in the number that cannot cross the experimental space. ( c ) The percentage of randomly placed static 'beads' inaccessible to diffusing ribozyme—a measure of system compartmentalization—rises steeply as a function of lattice blocks (means ± s.e.m., n =20). Full size image To investigate how such structures could affect replicase evolution, we extended the simulation to analyse the effect of parasites (replicated preferentially but unable to replicate themselves) on ribozyme replication. Degradation, diffusion and replication of replicases and interspersed parasites were modelled within a toroidal 'eutectic' lattice as Markov processes using Monte Carlo steps, as previously developed for chemical reaction analysis with single-molecule resolution [35] , [36] ( Fig. 8a ). Under most conditions, replication parasites, once introduced, quickly 'poisoned' replicase populations. Progressive disruption of lattice connectivity to the point previously found to lead to a drop in diffusive transport ( Fig. 7b ) now led to the emergence of stable replicase populations ( Fig. 8b ), even in the presence of excess ( Fig. 8c ) or rapidly diffusing parasites ( Fig. 8d ). Although both higher parasite/replicase ratios and faster parasite diffusion do reduce 'replicase success' (that is, the establishment of stable replicase populations within the lattice), in both cases the effect is attenuated as the number of lattice blocks and hence lattice fragmentation increases. At high levels of lattice fragmentation, the effects of both high numbers of parasites and faster parasite diffusion are effectively neutralized ( Fig. 8c,d ). In other words, although in an open lattice faster diffusing parasites are much more destructive, as lattice fragmentation and thus compartmentalization increases, parasite density and the speed of parasite diffusion become increasingly irrelevant, and the system as a whole becomes robustly resistant to parasite takeover. Thus, lattice fragmentation, as predicted from SEM imaging of eutectic phases formed from dilute starting solutions, recapitulates diffusion restriction and predicts the emergence of quasicellular compartmentalization capable of supporting replicase growth and evolution. 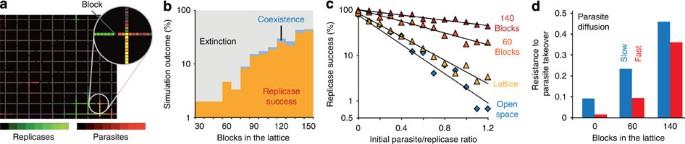Figure 8: Modelling of ribozyme diffusion and replication in the eutectic phase. (a) Replication and diffusion of parasites (red) and replicases (green) simulated within a lattice space (grey). Yellow represents equal numbers of replicases and parasites. The addition of blocks (black) to the channels of the grid-lattice decreased connectivity. (b) Simulation outcomes (after 20,000 time steps;n≥50). If blocks are <30, parasites invariably drove replicases to extinction under these simulation conditions. (c) The replicase success promoted by lattice blocks is maintained over a range of starting parasite/replicase ratios (n≥100) and is increasingly robust at higher lattice fragmentation (open space, blue diamonds; just lattice, yellow triangles; 60 blocks, orange triangles; 140 blocks, red triangles). (d) Resistance to parasite takeover (the relative chance of replicase success after introduction of one parasite per replicase) is less affected by a threefold increase in parasite diffusion speed (blue bars to red bars) when lattice fragmentation increases. Figure 8: Modelling of ribozyme diffusion and replication in the eutectic phase. ( a ) Replication and diffusion of parasites (red) and replicases (green) simulated within a lattice space (grey). Yellow represents equal numbers of replicases and parasites. The addition of blocks (black) to the channels of the grid-lattice decreased connectivity. ( b ) Simulation outcomes (after 20,000 time steps; n ≥50). If blocks are <30, parasites invariably drove replicases to extinction under these simulation conditions. ( c ) The replicase success promoted by lattice blocks is maintained over a range of starting parasite/replicase ratios ( n ≥100) and is increasingly robust at higher lattice fragmentation (open space, blue diamonds; just lattice, yellow triangles; 60 blocks, orange triangles; 140 blocks, red triangles). ( d ) Resistance to parasite takeover (the relative chance of replicase success after introduction of one parasite per replicase) is less affected by a threefold increase in parasite diffusion speed (blue bars to red bars) when lattice fragmentation increases. Full size image Formation of ice from dilute starting mixtures not only provides compartmentalization of RNA replication but also relieves its dependence on prebiotically implausible solute and substrate concentrations. Owing to the concentrating effect of eutectic phase formation, ribozyme-catalysed RNA replication can proceed from starting mixtures containing as little as 1 mM Mg 2+ and 10 μM ribonucleotide triphosphates. The strength of this concentration effect is inversely proportional to the total solute level [15] , [19] and consequently dependent on the salinity of the environment; it would therefore have been best realized in a freshwater environment. It is notable that other prebiotically relevant processes such as vesicle formation, concentration of solutes by thermophoresis and the non-enzymatic condensation of activated mononucleotides are also inhibited by saline environments [37] , [38] . Although low temperatures within the ice slow down enzymatic RNA polymerization, stabilization and reduced degradation of ribozyme replicase offset this effect, allowing replication to continue for weeks and yielding exceptionally long replication products of 32 nucleotides, approaching the size of small ribozymes. Although ice thus more than doubles the primer extension capability of the R18 RNA polymerase ribozyme [13] , significant further improvements are required to bring self-replication of the 195 nucleotide-long ribozyme within reach. While in-ice RNA replication activity may be enhanced further by continued fine-tuning of solute concentrations and identity, there is no denying that R18, in its current form, is maladapted to the ice phase. R18 was evolved at 22 °C [13] , and thus operates in ice at a temperature almost 30 °C below this. Adaptation of the ribozyme to low temperatures and the specific environment of the eutectic phase may best be achieved by directed evolution of ribozyme activity within the ice phase. We anticipate that ribozymes evolved this way would exhibit faster in-ice reaction rates while yielding prolonged activity because of the increased RNA stability at low temperatures. The latter may accelerate RNA evolution in other ways, such as by buffering the effects of destabilizing mutations on ribozyme structure and activity, thereby allowing higher levels of genetic drift and effectively increasing the error threshold at which an RNA replicase could operate [32] . Prebiotic RNA self-replication within eutectic ice phases presupposes the existence of significant bodies of ice on the surface of the primordial Earth. Previous assumptions that the surface and ocean temperatures on the Hadean Earth were high (Hadean (Greek: 'hellish')), and therefore incompatible with surface ice, have recently been challenged [39] , [40] , [41] , [42] . These studies all suggest temperate climatic conditions for the Hadean and Archean eons, compatible with substantial polar and seasonal ice deposits. Furthermore, subsequent planetary-wide crustal melt and 'sterilization' through the Late Heavy Bombardment has also been called into question [43] . Thus, water ice might have been present on the surface of the Earth ever since planetary formation. In conclusion, we show that the physicochemical properties of water ice, a chemically simple medium likely to have been widespread on the early Earth, as well as on planetary bodies in general [44] , [45] , can significantly enhance the efficiency of RNA-catalysed RNA replication without compromising its fidelity. Although protocellular compartmentalization can take many forms [11] , it is often considered that RNA self-replication originated within membraneous protocellular vesicles in an ambient, aqueous environment [9] , [46] . Here, we demonstrate that neither RNA replication nor compartmentalization is necessarily confined to the solution phase, or indeed to ambient temperatures, but that both are provided within the aqueous eutectic phase of water ice at subzero temperatures. Ice had previously been shown to stabilize nucleotide precursors [47] , [48] and catalyse both the de novo and templated synthesis of random RNA oligomers [16] , [17] , [18] , [49] . Our results imply a potentially wider role for ice, promoting all the steps from prebiotic oligomer synthesis to the emergence of RNA self-replication and Darwinian evolution. In analogy to present day sympagic biota, ice might thus have harboured a 'cold RNA world' [19] , [50] , [51] , predating the emergence of membranous protocells. Ribozyme construct preparation The ribozyme polymerase gene was assembled by PCR from the following DNA oligonucleotides: 5′-GGAAAAAGACAAATCTGCCCTCAGAGCTTGAGAACATCTTCGGATGCAGAGGAGGCAGCCTCCGGTGGCG-3′, 5′-CCCGCCGAAGCGGGAGTATTGGGCGCCTGTTGAGAACGTTGGCGCTATCGCGCCACCGGAGGCTGCCTCCTCTGC-3′, 5′-CGCCCAATACTCCCGCTTCGGCGGGTGGGGATAACACCTGACGAAAAGGCGATGTTAGACACGCCAAGGT-3′ and 5′-GGAGCCGAAGCTCCGGGGATTATGACCTTGGCGTGTCTAACATCGCCTT-3′. Cloning and sequencing yielded a plasmid containing the expected sequence, which was used to generate a PCR product consisting of a T7 promoter sequence upstream of the ribozyme construct sequence: 5′-GGACAACCAAAAAGACAAATCTGCCCTCAGAGCTTGAGAACATCTTCGGATGCAGAGGAGGCAGCCTCCGGT GGCGCGATAGCGCCAACGTTCTCAACAGGCGCCCAATACTCCCGCTTCGGCGGGTGGGGATAACACCTGAC GAAAAGGCGATGTTAGACACGCCAAGGTCATAATCCCCGGAGCTTCGGCTCC-3′. The ribozyme sequence used is a variant of the Round 18 ribozyme [13] , with a lengthened 5′-terminus from the parental 18.12 construct (the presence of which did not affect ribozyme activity in the original study). Ribozyme was transcribed using Ambion MegaShortScript Kit, and purified with Qiagen RNeasy Mini Kit. Ribozyme used in assays always included an equimolar amount of 3′-dideoxy RNA 'stem' oligo (5′-GGCACCC-3′) to complete the construct. Polymerase assay To set up standard primer extension reactions, 10 pmol each of ribozyme construct, RNA template and 5′-fluorescein-labelled RNA primer were annealed in 1.3 μl of water (50 °C for 5 min, 17 °C for 10 min) and kept on ice before the addition of 38.7 μl of chilled extension buffer (f.c. 200 mM MgCl 2 , 50 mM Tris•HCl (pH 8.3), 4 mM of each ribonucleotide triphosphate). MgCl 2 was pretreated with Bio-Rad Chelex 100 resin to remove heavy metal ions. The 10-nucleotide RNA primer 5′-CUGCCAACCG-3′ was 5′-fluorescein modified to allow visualization of extension products. The ribozyme 5′ terminus could hybridize to the eight 3′ bases of the RNA capture template 5′-CAAUGAAUCCACGCUUCGCACGGUUGGCAGAACAGGUUGUCC-3′; these bases were absent in the 'free' RNA template. Longer RNA template sequences that, instead of 20, allowed 22 nucleotides (5′-GUCAAUGAAUCCACGCUUCGCACGGUUGGCAGAACAGGUUGUCC-3′) or 41 nucleotides (5′-GUCAAUGACACGCUUCGCACACGCUUCGCACACGCUUCGCACGGUUGGCAGAACAGGUUGUCC-3′) of templated extension were used in Figure 4a ; extensions with the 41-nucleotide template used 20 pmol of each RNA per reaction. Protein polymerase extension assays ( Fig. 1b , left panel) were set up as above with 'free' template, but T7 RNA polymerase (New England Biolabs) was added after buffer (f.c. 0.25 μM, in 1× T7 RNA polymerase buffer (New England Biolabs) supplemented with 14 mM MgCl 2 and 4 mM of each ribonucleotide triphosphate). To explore the influence on the extension of Mg 2+ counterions other than Cl − (SO 4 2− , Br − , NO 3 − , CH 3 CO 2 − ), the MgCl 2 in the extension buffer was replaced with equimolar concentrations of the relevant Mg salt. In-ice primer extensions were first frozen at −25 °C for 10 min, then transferred to a Techne RB-5 refrigerated bath, maintained at −7 °C by a Techne Tempette TE-8D thermostat. Omitting the freeze at −25 °C before the −7 °C incubation resulted in supercooled reactions that remained aqueous. Other methods to achieve ice formation—by flash-freezing the reaction in a mixture of ethanol and dry ice before incubation at −7 °C, or by adding an ice crystal to a supercooled reaction—yield eutectic ice phases supporting comparable levels of in-ice RNA replication. Reactions were stopped by 0.5 V of 0.5 M EDTA, heated for 5 min at 94 °C in 6 M urea with a 20× excess of competing RNA oligonucleotide (5′-CUGCCAACCGUGCGAAGCGUGGAUUCAUUG-3′ or, with the 41-nucleotide template, 5′-GGACAACCUGUUCUGCCAACCGUGCGAAGCGUGUGCGAAGCGUGUGCGAAGCGUGUCAUUGAC-3′), resolved by urea-PAGE and analysed using a Typhoon Trio scanner. Gel image brightness and contrast were adjusted to illustrate extension product banding patterns. Dilution assays To set up diluted extension reactions, 10 pmol each of ribozyme construct, template and primer were annealed as above. Extension buffer was diluted with water and chilled on ice before addition; for an n -fold dilution, ( n −1)×40 μl of water were added to the extension buffer. After incubation, reactions were stopped with 20 μl of 0.5 M EDTA; aliquots containing 1.5 pmol of primer were taken from each, made up to equal volumes with water, dried and analysed by PAGE as above. Primer extension quantification Primer extension was quantified using ImageQuant TL. Each gel image lane was divided up into bands corresponding to unextended primer and each extension product; an intensity value for each band was given by subtracting the bulk of the background signal (using a baseline drawn between intensity minima in the lane). Further background correction was then carried out by subtracting the intensity values of an empty lane, allowing the quantification of weak extensions. These corrected intensity values were used to calculate the average extension per primer in a lane ( E ) [8] : where x n is the intensity of the band corresponding to n base additions. Ribozyme degradation assay 5′-fluorescein-labelled ribozyme was transcribed using Ambion MegaShortScript Kit, in the presence of 3.75 mM each of ATP, UTP and CTP, 2 mM of GTP, and 2 mM of 5′-fluorescein-labelled AG RNA dinucleotide starter (Dharmacon), before purification using RNeasy Mini Kit. 3 pmol each of fluorescently labelled ribozyme, template and primer (without the fluorophore) were annealed together in 9 μl of water. A volume of 2.4 μl of 1 M MgCl 2 and 0.6 μl of 1 M Tris•HCl (pH 8.3) was chilled on ice and added to the RNAs before incubation at different temperatures and resolution as above. The ratio of full-length ribozyme to shorter fragments was determined, after comparison with starting samples to correct for the presence of premature transcription termination products. Sequencing of extended primers The indicated bands were excised from the gel, and the RNA was extracted, poly-A-tailed, reverse-transcribed and PCR-amplified to allow Illumina sequencing. Geometric means were calculated for all error rates. SEM Samples with the same composition as extension reactions or diluted extension reactions were loaded into the ends of 1 mm-diameter copper tubes, leaving a protruding drop of solution. After flash-freezing over liquid N 2 , samples were transferred to a Reichert AFS (Leica) at −7 °C and incubated for 60–100 min under a N 2 atmosphere to allow eutectic phase formation. At the end of the incubation, to preserve eutectic phase structure, samples were transferred using chilled tweezers directly to liquid N 2 , in which they were mounted on a transfer shuttle and moved to a PP2000 Cryo-SEM preparation chamber (Quorum) at −130 °C. The sample was freeze-fractured at the neck of the tube, and the temperature was raised (−90 °C for 10 min for Figs. 2b and 5d , −80 °C for 30 min for Fig. 6b , −85 °C for 15 min for Fig. 6c,d ) to allow sublimation of water from ice crystals, leaving the salts of the eutectic phase protruding. Longer sublimations at higher temperatures led to more water loss, exposing more extensive eutectic phase structures. On cooling and sputter coating with ∼ 30 nm of gold, images were acquired using an FEI XL30 FEG SEM. Ribozyme diffusion assay Primer extension on 1 μm-diameter streptavidincoated beads (MyOne, Dynal) was detected in a manner similar to that described for BEAMing Up [52] . DNA products were stained with Picogreen (Invitrogen), and bead populations were analysed on a FACSCalibur instrument (BD Biosciences) with an FL-1 detector voltage of 450 V; typically, about 20,000 sorting events corresponding to single beads (as gated by event forward and side scatter) were collected per sample. Flow cytometry data were analysed using FlowJo software (TreeStar). Positive beads (that encountered the ribozyme) were defined as those with a fluorescence signal >30.5. A background level of 0–3% positive beads was also observed in pure water ice columns, presumably from localized small-scale thawing of the top of the column on ribozyme addition. Correcting for this, Figure 5c displays the percentage of the remaining beads that are extended. How to cite this article: Attwater, J. et al . Ice as a protocellular medium for RNA replication. Nat. Commun. 1:76 doi: 10.1038/ncomms1076 (2010).